Water enables mild oxidation of methane to methanol on gold single-atom catalysts As a 100% atom-economy process, direct oxidation of methane into methanol remains as a grand challenge due to the dilemma between activation of methane and over-oxidation of methanol. Here, we report that water enabled mild oxidation of methane into methanol with >99% selectivity over Au single atoms on black phosphorus (Au 1 /BP) nanosheets under light irradiation. The mass activity of Au 1 /BP nanosheets reached 113.5 μmol g catal −1 in water pressured with 33 bar of mixed gas (CH 4 :O 2 = 10:1) at 90 °C under light irradiation (1.2 W), while the activation energy was 43.4 kJ mol −1 . Mechanistic studies revealed that water assisted the activation of O 2 to generate reactive hydroxyl groups and •OH radicals under light irradiation. Hydroxyl groups reacted with methane at Au single atoms to form water and CH 3 * species, followed by oxidation of CH 3 * via •OH radicals into methanol. Considering the recycling of water during the whole process, we can also regard water as a catalyst. Advances in hydraulic fracturing technology have enabled ongoing discovery of large reserves of natural gas, which primarily contains methane [1] . At present, most of produced methane is burned for heating, transport, and electricity-generation purposes. Meanwhile, methane is the second most relevant greenhouse gas emitted from anthropogenic activities, as global warming potential of methane is 25 times higher than that of CO 2 [2] . In this case, it is highly desired to develop efficient techniques for upgrading of methane. The current industrial route is via steam or dry reforming to generate syngas (a mixture of CO and H 2 ), followed by Fischer–Tropsch synthesis or methanol synthesis [3] , [4] . Such route operated at high temperature (>700 °C) not only needs huge energy input, but also leads to the deactivation of catalysts because of coking [5] . Direct conversion of methane into chemicals or liquid fuels has been achieved under mild conditions [6] , [7] , [8] , [9] . For instance, aqueous Au-Pd colloids achieved selective oxidation of methane into methanol with H 2 O 2 as an oxidant under 30 bar of CH 4 at 50 °C [10] . Methane was reported to be oxidized into methanesulfonic acid by SO 3 over an electrophilic initiator at 50 °C [11] . However, these processes generally involve corrosive oxidant or expensive media, such as H 2 O 2 , oleum, trifluoroacetic acid, and hydrobromic acid, which is not suitable for commercialization [12] , [13] , [14] , [15] . Among direct processes, aerobic oxidation of methane into methanol is an ideal reaction with 100% atom economy (Eq. 1 ). The dilemma lies in activation of methane and over-oxidation of methanol [16] , [17] , [18] . Methane takes a non-polar tetrahedral structure with high dissociation energy of C–H bond (439.3 kJ mol −1 ), rendering great difficulties for activation [19] , [20] , [21] . As methane and O 2 are in singlet and triplet ground states, respectively, the direct reaction of methane with O 2 in ground states is spin-prohibition, which should be overcome [22] . Once methane is activated, the produced methanol tends to be over-oxidized into CO or CO 2 from a thermodynamic perspective (Eqs. 1 – 3 ) [23] . Therefore, it is important but challenging to achieve highly selective oxidation of methane with O 2 into methanol under ambient conditions. CH_4 + 0.5O_2 = CH_3OH    ΔH_298K = - 126.4kJ mol^ - 1
 (1) 
    CH_4 + 1.5O_2 = CO + 2H_2O    ΔH_298K = - 519.6kJ mol^ - 1
 (2) 
    CH_4 + 2O_2 = CO_2 + 2H_2O    ΔH_298K = - 802.6kJmol^ - 1
 (3) Herein, we achieved mild oxidation of methane into methanol over Au single atoms on black phosphorus (Au 1 /BP) nanosheets with the help of water under light irradiation. Photocatalysis offers an efficient approach to drive thermodynamically non-spontaneous reactions under mild conditions [24] , [25] . We applied black phosphorus (BP) nanosheets as the support that affords broadband solar absorption for photocatalysis [26] , [27] . During methane oxidation, the mass activity of Au 1 /BP nanosheets was 113.5 μmol g catal −1 in water pressured with 33 bar of mixed gas (CH 4 :O 2 = 10:1) at 90 °C under light irradiation (1.2 W). The selectivity for methanol reached as high as >99%. Based on mechanistic studies, water and O 2 were activated on Au 1 /BP nanosheets to form reactive hydroxyl groups and •OH radicals under light irradiation. The reactive hydroxyl groups enabled mild oxidation of methane into CH 3 * species, followed by oxidation of CH 3 * via •OH radicals into methanol. As water is consumed to form hydroxyl groups and produced via reaction of hydroxyl groups with methane, water is completely recycled and thus can also be regarded as a catalyst. Synthesis and characterizations of Au 1 /BP nanosheets To prepare Au 1 /BP nanosheets, we first synthesized bulk BP through a low-pressure transport route according to the reported literature [28] . BP nanosheets were prepared by liquid exfoliation of bulk BP. The diameter of free-standing BP nanosheets was several hundred nanometers (Supplementary Fig. 1 ). As measured by atomic force microscopy, the thickness of the as-obtained nanosheet was ca. 3.0 nm (Supplementary Fig. 2 ). We prepared Au 1 /BP nanosheets by injecting HAuCl 4 solution into a mixture containing ethanol and BP nanosheets with the use of a syringe pump under nitrogen protection. 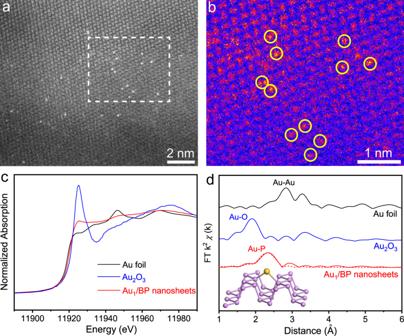Fig. 1: Structural characterizations of Au1/BP nanosheets. aHAADF-STEM image of Au1/BP nanosheets.bMagnified HAADF-STEM image with color-coded intensity. This image shows the region marked by dash box ina.cXANES spectrum anddEXAFS spectrum of Au1/BP nanosheets. Au foil and Au2O3were used as the references. The inset image indis a structural model of Au1/BP nanosheets. Violet and yellow spheres represent for P and Au atoms, respectively. Figure 1a shows a high-angle annular dark-field scanning transmission electron microscopy (HAADF-STEM) image of Au 1 /BP nanosheets, where the Au mass loading was determined as 0.2 wt%. The magnified HAADF-STEM image and its corresponding color-coded intensity map were shown in Fig. 1b , indicating the isolated distribution of Au atoms in the absence of Au nanoparticles (NPs). This point was further verified by HAADF-STEM images with lower magnifications (Supplementary Fig. 3 ). By increasing the concentration of HAuCl 4 solution, we obtained Au NPs on BP nanosheets (denoted as Au NPs/BP nanosheets). As shown in Supplementary Figure 4 , Au NPs with an average size of 6 nm were uniformly dispersed on BP nanosheets with a mass loading of 1.0 wt%. Fig. 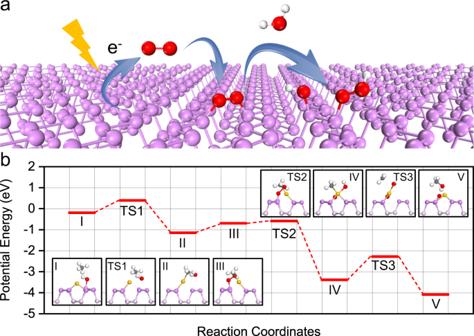Fig. 4: DFT studies. aSchematic illustration of oxygen activation on BP nanosheets.bReaction path for partial oxidation of methane over Au1/BP nanosheets under light irradiation. The inset images show the side views of the configurations. Yellow, violet, pink, red, gray, and white spheres represent Au, surface P, subsurface P, O, C, and H atoms, respectively. 1: Structural characterizations of Au 1 /BP nanosheets. a HAADF-STEM image of Au 1 /BP nanosheets. b Magnified HAADF-STEM image with color-coded intensity. This image shows the region marked by dash box in a . c XANES spectrum and d EXAFS spectrum of Au 1 /BP nanosheets. Au foil and Au 2 O 3 were used as the references. The inset image in d is a structural model of Au 1 /BP nanosheets. Violet and yellow spheres represent for P and Au atoms, respectively. Full size image We further characterized the global structure of Au 1 /BP nanosheets. X-ray diffraction (XRD) patterns revealed that both BP and Au 1 /BP nanosheets were well indexed to the orthorhombic phase of BP (Supplementary Fig. 5 ). Especially, two intense diffraction peaks at 34.2° and 52.3° corresponded to (040) and (060) facets of orthorhombic BP, respectively, which are representative layered planes of BP. No patterns corresponding to Au phase were observed, in concert with the isolated dispersion of Au atoms. Raman spectra of BP and Au 1 /BP nanosheets show similar peaks located at 361, 438, and 466 cm −1 , which were assigned to A g 1 (out-of-plane), B 2g , (in-plane), and A g 2 (in-plane) vibration modes of BP, respectively (Supplementary Fig. 6 ). To further determine the local environment in Au 1 /BP nanosheets, we measured X-ray absorption near-edge spectroscopy (XANES) and extended X-ray absorption fine structure (EXAFS). The Au L 3 -edge XANES profiles indicated that the Au species in Au 1 /BP nanosheets were in a mediate oxidation state (Fig. 1c ), according to the mediate intensity for white line compared with Au foil and Au 2 O 3 . As shown in EXAFS in R space (Fig. 1d ), the spectrum of Au 1 /BP nanosheets exhibited a prominent peak at 2.33 Å from the Au–P shell with a coordination number ( CN ) of 2.0 (Supplementary Table 1 ). No other typical peaks for Au–Au contribution at longer distances (>2.5 Å) or for Au–O contributions at shorter distance (<1.9 Å) were observed, revealing the isolated dispersion of Au atoms. The peak from the Au-Cl shell was not observed in XAFS spectra, indicating that residual Cl from the synthesis was absent on Au 1 /BP nanosheets. This result was also supported by the high-resolution X-ray photoelectron spectroscopy (XPS) spectrum which showed no signals for Cl (Supplementary Fig. 7 ). Further density functional theory (DFT) calculations were performed to establish the atomic model of Au 1 /BP nanosheets. To simulate Au 1 /BP nanosheets, we situated the Au single atom at the bridge P sites (inset of Fig. 1d ), considering thermodynamic stability and two Au–P bonds as revealed by EXAFS. To explore the band structure of BP and Au 1 /BP nanosheets, we conducted measurements of ultraviolet-visible-near infrared (UV-vis-NIR) absorption and valence XPS. From UV-vis-NIR spectra and the corresponding Tauc plots, the bandgaps of BP and Au 1 /BP nanosheets were 1.45 eV (Supplementary Fig. 8a , b). Mott–Schottky plots showed that the flat band potentials of BP and Au 1 /BP nanosheets were both –0.35 V (vs RHE) (Supplementary Fig. 8c ). According to valence XPS spectra, the valence band energy levels of BP and Au 1 /BP nanosheets were estimated as 1.35 and 1.31 eV below the Fermi level, respectively (Supplementary Fig. 8d ). Based on UV-vis-NIR absorption and valence XPS spectra, the complete band structure of Au 1 /BP nanosheets was obtained, similar to that of BP nanosheets (Supplementary Fig. 8e ). Therefore, the deposition of Au atoms on BP nanosheets led to negligible variation in the band structures of BP nanosheets. For comparison, we prepared Pt, Pd, and Rh single atoms/NPs on BP nanosheets, which were denoted as Pt 1 /BP, Pd 1 /BP, Rh 1 /BP, Pt NPs/BP, Pd NPs/BP, Rh NPs/BP nanosheets, respectively (Supplementary Figs. 9 and 10 ). The loading amounts of metal single atoms and NPs were controlled as 0.2 wt% and 1.0 wt%, respectively. The dispersion of metal species in these samples was further verified by diffuse reflectance infrared Fourier transform spectroscopy (DRIFTS) experiments using CO as a probe molecule. 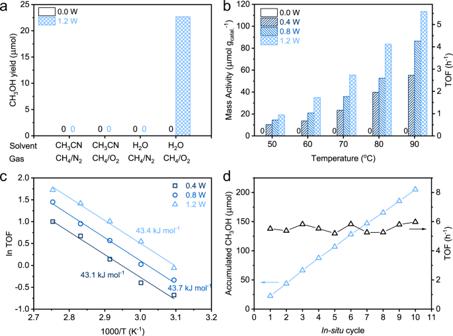Especially, DRIFTS spectra of M 1 /BP (M = Pt, Pd, and Rh) nanosheets only showed the peaks for the linear adsorption of CO, whereas, besides the peaks for the linear adsorption, the peaks for the bridge adsorption were also observed for M NPs/BP nanosheets (Supplementary Fig. Fig. 2: Catalytic performance of Au1/BP nanosheets in partial oxidation of methane. aComparison of methanol yields under different solvents and reactants at 90°C for 2 h.bMass activities and TOF numbers in 20 mL of water under 33 bar (CH4:O2= 10:1) at different temperatures under different light powers with an irradiation area of 3.14 cm2.cThe Arrhenius plots of Au1/BP nanosheets under different light intensities.dProducts and TOF numbers obtained by conducting in situ cycles. For each cycle, the catalytic reaction was operated under 33 bar (CH4:O2= 10:1) at 90°C for 2 h (1.2 W). 11 and Table 2 ). Catalytic properties of Au 1 /BP nanosheets towards partial oxidation of methane The catalytic tests were conducted in a slurry reactor with a sapphire window, which allowed the incidence of light from Xe lamp into the reactor to participate in the reaction (Supplementary Fig. 12 ). For a standard condition, the reaction was operated in 20 mL of water pressured with 33 bar of mixed gas (CH 4 :O 2 = 10:1) at 90 °C under light irradiation with a light power of 1.2 W and irradiation area of 3.14 cm 2 . For BP nanosheets, the product after 2 h was below detection limit. As for Au 1 /BP nanosheets, 22.7 μmol of methanol was generated without any by-products after 2 h (Fig. 2a ). Under the standard condition, the mass activity of Au 1 /BP nanosheets was 113.5 μmol g catal −1 , whereas the turnover frequency (TOF) number was 5.6 h −1 . Notably, the TOF number of Au 1 /BP nanosheets was higher than those of Au NPs/BP, M 1 /BP, and M NPs/BP (M = Pt, Rh, and Pd) nanosheets (Supplementary Fig. 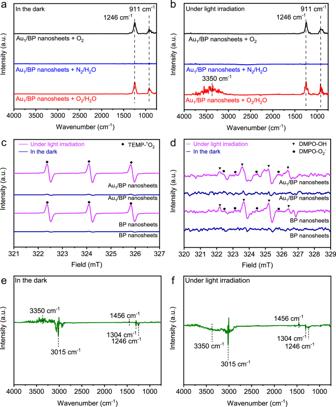13 ). Fig. 3: Mechanistic studies. In situ DRIFTS spectra of Au1/BP nanosheets purged by 1 bar of different gases at 90°C (a) in the dark and (b) under light irradiation. Background spectra were acquired after flowing under 1 bar of N2with the rate of 20 sccm at 150°C for 0.5 h, followed by cooling to 90°C.cIn situ ESR spectra of BP and Au1/BP nanosheets under different conditions in the presence of TEMP.dIn situ ESR spectra of BP and Au1/BP nanosheets under different conditions in the presence of DMPO. In situ DRIFTS spectra of Au1/BP nanosheets purged by 1 bar of CH4at 90°C (e) in the dark and (f) under light irradiation. Catalysts were purged by 1 bar of O2/H2O at 90°C for 0.5 h, followed by 1 bar of N2at 150°C for 0.5 h. Afterwards, the catalysts were purged by 1 bar of CH4at 25°C for 0.5 h to obtain background spectra. The TOF number of Au 1 /BP nanosheets was comparable to that of the state-of-the-art catalysts under similar reaction conditions (Supplementary Table 3 ). When we removed light irradiation from the standard condition, the product was below detection limit (Fig. 2a ). As such, light irradiation helped drive the formation of methanol. Fig. 2: Catalytic performance of Au 1 /BP nanosheets in partial oxidation of methane. a Comparison of methanol yields under different solvents and reactants at 90°C for 2 h. b Mass activities and TOF numbers in 20 mL of water under 33 bar (CH 4 :O 2 = 10:1) at different temperatures under different light powers with an irradiation area of 3.14 cm 2 . c The Arrhenius plots of Au 1 /BP nanosheets under different light intensities. d Products and TOF numbers obtained by conducting in situ cycles. For each cycle, the catalytic reaction was operated under 33 bar (CH 4 :O 2 = 10:1) at 90°C for 2 h (1.2 W). Full size image To further investigate the influence of light irradiation, we varied the light powers from 0.4 to 1.2 W. As shown in Fig. 2b and Supplementary Figure 14 , the activity of Au 1 /BP nanosheets increased with the rise of light intensity at the same temperature. Notably, the activation energy ( E a ) of Au 1 /BP nanosheets was almost independent of light intensity (Fig. 2c ). Especially, E a of Au 1 /BP nanosheets at the power of 1.2 W was 43.4 kJ mol −1 , approaching to that (43.7 kJ mol −1 ) at 0.8 W and that (43.1 kJ mol −1 ) at 0.4 W (Fig. 2c ). In addition, the reaction was determined as heterogeneous instead of homogeneous, because the use of the supernate after the reaction, HAuCl 4 -H 3 PO 4 , and Au(OH) 3 -H 3 PO 4 as the catalysts gave rise to trace amounts of products (Supplementary Fig. 15 ). Moreover, we evaluated the wavelength-dependent apparent quantum yields (AQYs) of methanol. A high AQY of 17.4% was obtained under the irradiation of monochromatic light at 350 nm (Supplementary Fig. 16 ). We further explored the influence of the solvent and reactants during partial oxidation of methane. Substitution of water with acetonitrile as the solvent from the standard condition gave rise to no products (Fig. 2a ). In this case, water enables mild oxidation of methane under light irradiation. When O 2 was replaced by N 2 from the standard condition, leaving water as the oxidant, no detectable product was observed (Fig. 2a ). As such, O 2 was an indispensable oxidant, whereas only water was unable to oxidize methane under such mild reaction. In order to investigate the dependence of catalytic performance on reactants, we varied the partial pressures of CH 4 and O 2 at 90 °C under light irradiation. Increasing CH 4 partial pressure led to the rise of conversion while keeping the selectivity for methanol above 99% (Supplementary Fig. 17a ). Increasing O 2 partial pressure also increased the conversion and lowered the selectivity for methanol with the production of CO 2 (Supplementary Fig. 17b ). To determine whether the reaction was limited by mass transfer, we varied the stirring rates and the volumes of water. Despite of the varied stirring rates and the volumes of water, the mass activity still kept almost unchanged, indicating that the reaction kinetics was not determined by diffusion (Supplementary Fig. 18 ). When we used methanol as the reactants over Au 1 /BP nanosheets under light irradiation and 33 bar (N 2 :O 2 = 10:1) at 90 °C, the conversion of methanol was below detection limit. In this case, Au 1 /BP nanosheets were unable to catalyze the oxidation of methanol under such reaction conditions, indicating the high intrinsic selectivity for methanol. To investigate stability of the catalysts, we tested Au 1 /BP nanosheets for successive in situ cycles of reaction, where catalysts were not removed from the reaction during the whole test. For each cycle, the catalytic reaction proceeded under standard conditions for 2 h. After 10 in situ cycles (20 h in total), about 205.2 μmol of methanol was generated in total with the fluctuation of TOF below 7% (Fig. 2d ). Moreover, the atomic dispersion of Au was still maintained after 10 in situ cycles, where only Au–P bonds were observed in the absence of Au–Au bonds or Au–O bonds (Supplementary Fig. 19 and Table 1 ). Mechanistic insights into the activation of O 2 In order to investigate how water promotes methane oxidation under light irradiation, we conducted in situ DRIFTS measurements. Background spectra were acquired after flowing with 1 bar of N 2 at 150 °C for 0.5 h, followed by cooling to 90 °C. In situ DRIFTS spectrum of Au 1 /BP nanosheets after the treatment with O 2 in the dark at 90 °C showed two peaks at 1246 and 911 cm −1 , which were assigned to the stretching vibrations of P=O and P–O–P bonds, respectively (Fig. 3a ). The assignment of the peaks was supported by DFT calculations, reported literature, and isotope-labeling DRIFTS measurements (Supplementary Table 4 and Fig. 20 ). The peaks for P=O and P–O–P bonds were also observed when Au 1 /BP nanosheets were purged by O 2 under light irradiation (1.2 W) at 90 °C (Fig. 3b ). To simulate the reaction condition in the presence of water, N 2 was allowed to bubble in deionized water, followed by flowing into the cell, in order to bring the saturated water vapor into the cell, denoted as the treatment of N 2 /H 2 O. Under the atmosphere of N 2 /H 2 O, no peaks were observed, whenever in the dark or under light irradiation (Fig. 3a, b). As such, O 2 enabled the oxidization of BP nanosheets, whereas only H 2 O interacted weakly with the catalyst. Compared with the circumstances of O 2 , the mixture of O 2 /H 2 O made negligible differences in the dark, but gave rise to a new peak at 3350 cm −1 for the stretching vibration of hydroxyl groups under light irradiation (Fig. 3 a, b). In this case, water reacted with O 2 over Au 1 /BP nanosheets under light irradiation, resulting in the formation of hydroxyl groups. Fig. 3: Mechanistic studies. In situ DRIFTS spectra of Au 1 /BP nanosheets purged by 1 bar of different gases at 90°C ( a ) in the dark and ( b ) under light irradiation. Background spectra were acquired after flowing under 1 bar of N 2 with the rate of 20 sccm at 150°C for 0.5 h, followed by cooling to 90°C. c In situ ESR spectra of BP and Au 1 /BP nanosheets under different conditions in the presence of TEMP. d In situ ESR spectra of BP and Au 1 /BP nanosheets under different conditions in the presence of DMPO. In situ DRIFTS spectra of Au 1 /BP nanosheets purged by 1 bar of CH 4 at 90°C ( e ) in the dark and ( f ) under light irradiation. Catalysts were purged by 1 bar of O 2 /H 2 O at 90°C for 0.5 h, followed by 1 bar of N 2 at 150°C for 0.5 h. Afterwards, the catalysts were purged by 1 bar of CH 4 at 25°C for 0.5 h to obtain background spectra. Full size image We further explored whether hydroxyl groups were bonded with P atoms or Au atoms. We conducted quasi situ XPS measurements after the treatment of Au 1 /BP nanosheets with O 2 /H 2 O mixed gas in the dark or under light irradiation at 90 °C. O 1 s spectra confirmed that P–O–P and P=O bonds were formed in the dark, whereas P–OH bonds were generated under light irradiation (Supplementary Fig. 21a ). Whenever Au 1 /BP nanosheets were treated with O 2 /H 2 O in the dark or under light irradiation, Au 4 f spectra showed negligible difference compared with that without any treatment (Supplementary Fig. 21b ). In this case, Au atoms were not further oxidized by O 2 /H 2 O in terms of the coordination with oxygen-containing groups such as O atoms or hydroxyl groups. To further verify this point, we conducted 1 H solid nuclear magnetic resonance (NMR) measurements with the reference of Au(OH) 3 . After the treatment of Au 1 /BP nanosheets with O 2 /H 2 O under light irradiation, magic angle spinning (MAS) NMR spectrum showed no detectable signals (Supplementary Fig. 22 ), excluding the possibility of the adsorption of hydroxyl groups on Au atoms. Therefore, hydroxyl groups were adsorbed on P atoms, generating P–OH ensembles. Considering the short lifetime of photo-induced radicals that cannot be detected by in situ DRIFTS or quasi situ XPS, we conducted measurements of in situ electron spin resonance (ESR) spectroscopy using different trapping agents. 2,2,6,6-tetramethylpiperidine (TEMP) was selected to detect singlet O 2 ( 1 O 2 ), while 5,5-dimethyl-1-pyrroline-N-oxide (DMPO) was selected for the detection of superoxide ions (O 2 − ) and hydroxyl radicals (•OH). As illustrated in Figure 3c , d, signals for 1 O 2 , O 2 − , and •OH were all observed for both BP and Au 1 /BP nanosheets under light irradiation. Collectively, the water-promoted activation of O 2 under light irradiation involves the formation of 1 O 2 , O 2 − , •OH, and P–OH species. We carried out DFT calculations to determine the adsorption configurations of dissociated O atoms or hydroxyl groups on Au 1 /BP nanosheets. The optimized configurations were obtained according to thermodynamic consideration. Supplementary Figure 23 shows the optimized adsorption configuration of two O atoms on Au 1 /BP nanosheets. Especially, one O atom (O1) is located at the top P atom to form a P=O ensemble. The other O atom (O 2 ) at the groove site is linked to two P atoms to form a P–O–P ensemble. These two ensembles were both observed in in situ DRIFTS spectrum (Fig. 3a ). As such, the activation of O 2 in the dark follows Eq. 4 . O_2 + 3P→P = O + P - O - P
 (4) Figure 4a shows the activation of O 2 under light irradiation (Supplementary Fig. 24 ). Especially, the electrons from the valence band of BP are excited by light irradiation to react with O 2 at the triplet ground states ( 3 O 2 ), resulting in the formation of O 2 − (Eq. 5 ). O 2 − recombines the photo-generated holes to form the excited O 2 at the singlet states, 1 O 2 (Eq. 6 ). 1 O 2 reacts with H 2 O to yield OH * and HOO * which can be split into •OH radicals (Eqs. 7 and 8 ). ^3O_2 + e^ -→O_2^ -
 (5) 
    O_2^ - + h^ + → ^1O_2
 (6) 
    ^1O_2 + H_2O→HOO^ ∗ + OH^ ∗
 (7) 
    HOO^ ∗→∙ OH + O^ ∗
 (8) Fig. 4: DFT studies. a Schematic illustration of oxygen activation on BP nanosheets. b Reaction path for partial oxidation of methane over Au 1 /BP nanosheets under light irradiation. The inset images show the side views of the configurations. Yellow, violet, pink, red, gray, and white spheres represent Au, surface P, subsurface P, O, C, and H atoms, respectively. Full size image Mechanistic insights into the oxidation of CH 4 To reveal the role played by P–OH ensembles, we carried out in situ DRIFTS measurements of Au 1 /BP nanosheets under CH 4 after forming hydroxyl groups or not. Especially, the catalyst was purged by 1 bar of O 2 /H 2 O at 90 °C for 0.5 h in the dark to generate P=O and P–O–P ensembles, or under light irradiation to yield P=O, P–O–P, and P–OH ensembles. Afterwards, the catalyst was purged by 1 bar of CH 4 at 25 °C for 0.5 h to obtain background spectra. In situ DRIFTS spectra were recorded with CH 4 flow at 90 °C in the dark or under light irradiation. Notably, in in situ DRIFTS spectra, upward peaks correspond to newly appeared species, whereas downward peaks correspond to the loss of existed species. When both the pre-treatment and in situ DRIFTS measurements were conducted in the dark, both upward and downward peaks were observed (Fig. 3e ). Upward peaks included that at 3350 cm −1 for P–OH ensembles and that at 1456 cm −1 for CH 3 * . Downward peaks included those at 3015 and 1304 cm −1 for CH 4 * , and that at 1246 cm −1 for P=O ensembles. As such, P–OH and CH 3 * was generated, whereas P=O ensembles and CH 4 * were consumed. We propose that the reaction occurred as Eq. 9 . CH_4^ ∗ + P = O→CH_3^ ∗ + P - OH
 (9) Considering the absence of products in the dark, CH 3 * was unable to be further oxidized into methanol under mild condition in the dark. In other words, partial dehydrogenation of methane yielded inert P–OH ensembles. When both the pre-treatment and in situ DRIFTS measurements were conducted under light irradiation, the downward peaks comprised those for P–OH ensembles, P=O ensembles, and CH 4 * , whereas the upward peak only contained that for CH 3 * (Fig. 3f ). Considering methanol production under light irradiation, such reactive P–OH ensembles allowed mild oxidation of methane into CH 3 * and methanol in sequence. In addition, the in situ DRIFTS spectrum recorded in the dark after the pre-treatment under light irradiation was similar to Fig. 3f (Supplementary Fig. 25 ). To further identify how P–OH ensembles participated in the reaction, we combined temperature-programmed surface reaction with mass spectroscopy (TPSR-MS) using an isotope label. Especially, we used 18 O-labeled water (H 2 18 O) and routine O 2 ( 32 O 2 ) to pre-treat the catalyst in the dark or under light irradiation. TPSR-MS measurements were operated in the dark under CH 4 when the temperature rose from 50 to 300 °C. For pre-treatment in the dark, all the products were below the detection limit (Supplementary Fig. 26a , b). With regard to pre-treatment under light irradiation, four types of products were detected, including CH 3 18 OH, CH 3 16 OH, H 2 18 O, and H 2 16 O (Supplementary Fig. 26c ). Moreover, no peaks for CO 2 were observed, indicating the high selectivity for methanol (Supplementary Fig. 26d ). Notably, the temperature (above 200 °C) for methanol production was much higher than that (90 °C) during catalytic tests under light irradiation, because TPSR was conducted in the dark. In other words, methane oxidation under light irradiation follows a different path from that in the dark, despite O 2 activation under light irradiation. To investigate the mechanisms of methane oxidation under different conditions, we conducted DFT calculations. When both O 2 activation and CH 4 oxidation proceed in the dark, CH 4 dissociates into CH 3 * bonded to an Au atom and H * stabilized by a P=O ensemble to form a P–OH ensemble (Supplementary Fig. 27 ). The reaction of P–OH with CH 3 * exhibits an energy difference between configurations II and TS3 of 2.18 eV, which is much higher than that (0.42 eV, configurations II → TS1) of the recombination of CH 3 * and H * into CH 4 (Supplementary Fig. 27 ). The apparent energy barrier is defined as the energy difference between the initial state and the transition state with the highest energy. In this case, the apparent energy barrier (configurations I → TS3) is 2.62 eV for the conversion of CH 4 into CH 3 OH. Therefore, in the dark, P–OH ensembles cannot afford further oxidation of CH 3 * into methanol over Au 1 /BP nanosheets, though both O 2 and CH 4 can be activated. After the activation of O 2 under light irradiation, we consider the oxidation of CH 4 in the dark. The lack of continuous light leads to the adsorption of •OH into hydroxyl groups. Once two reactive hydroxyl groups are formed, one hydroxyl group reacts with CH 4 to generate CH 3 * and water. This step is the most thermodynamically favorable among different routes of CH 4 activation, exhibiting an energy barrier of 0.58 eV (Supplementary Table 5 and Fig. 28 , configurations I → TS1). Afterwards, the other hydroxyl group migrates from P atom to Au atom for further oxidation of CH 3 * (Supplementary Fig. 28 , configurations III → TS2 → IV). The last step is the integration of hydroxyl groups and CH 3 * to form methanol (Supplementary Fig. 28 , configurations IV → TS3 → V). The barrier of this step is 1.15 eV, thus determined as the rate-limiting step. Notably, the energy difference between configurations III and TS3 is as large as 1.67 eV (Supplementary Fig. 28 ). The apparent energy barrier (configurations I → TS3) is 1.03 eV for the conversion of CH 4 into CH 3 OH (Supplementary Fig. 28 ). We further focused on the reaction channel when both O 2 activation and CH 4 oxidation proceed under light irradiation. Upon the activation of O 2 , the generated hydroxyl group reacts with CH 4 to form water and CH 3 * stabilized by an Au atom (Fig. 4b ). The breakage of O–O bond in HOO * generates •OH which further co-adsorbs and reacts with CH 3 * on the Au atom, exhibiting an energy barrier as low as 0.25 eV (Fig. 4b , configurations III → TS2). Methanol is produced by the combination of OH * and CH 3 * on the Au atom with the energy barrier of 1.10 eV, which is determined as the rate-limiting step (Fig. 4b , configurations IV → TS3 → V). Notably, the remaining oxygen atoms on Au 1 /BP nanosheets are also able to activate CH 4 at 90 °C with the energy barrier of 1.19 eV, so as to complete the reaction cycle (Supplementary Fig. 29 ). Moreover, the apparent energy barrier for CH 4 conversion into CH 3 OH under light irradiation (Fig. 4b , configurations I → TS1) is only 0.58 eV, much lower than that (1.03 eV) in the dark. These results explain that 90 °C enables the oxidation of methane into methanol during catalytic tests under light irradiation, whereas methanol was produced above 200 °C during TPSR-MS experiments after the pre-treatment under light irradiation. To explain the high selectivity for methanol, we investigated the processes of CH 4 dehydrogenation and methanol oxidation. Except for CH 4 dehydrogenation into CH 3 * , the other dehydrogenation steps (CH x * → CH x−1 * + H * , x = 1, 2, 3) are all highly endothermic (Supplementary Fig. 30 ). In this case, the Au atom stabilizes CH 3 * to prevent deeper dehydrogenation. Moreover, we weighed the energy barriers for methanol oxidation, methanol desorption, and methane activation. Especially, the energy barrier for methanol oxidation by P–OH species is 1.31 eV, which is higher than that (apparent energy barrier, 0.58 eV) for methane activation and that (0.90 eV) for methanol desorption (Supplementary Fig. 31 ). Similar case also applies to P=O species where the energy barriers for methanol oxidation and desorption are 1.82 and 0.83 eV, respectively (Supplementary Fig. 31 ). As such, the produced methanol tends to desorb from the catalyst surface and dissolve in water instead of further oxidation under mild conditions such as 90 °C and 3 bar of O 2 partial pressure. Moreover, considering the low concentration of the produced methanol and the stabilization of methanol by the polar solvent of water, the dissolved methanol is unlikely to re-adsorb on the catalyst surface for further oxidation. In conclusion, we demonstrated that water enabled mild oxidation of methane into methanol with >99% selectivity over Au 1 /BP nanosheets under light irradiation. We found that water and O 2 reacted under light irradiation to generate reactive hydroxyl groups and •OH radicals. Hydroxyl groups reacted with methane at Au single atoms to form water and CH 3 * species. CH 3 * species were further oxidized by •OH radicals to generate methanol. As water is completely recycled during the whole process, it can also be regarded as a catalyst. Our findings shed light on insights into the role played by water during methane oxidation. Moreover, this work offers an effective strategy for upgrading methane at ambient condition suitable for local, on-site applications. Catalyst preparation In all, 500 mg of red phosphorus, 20 mg of Sn, and 10 mg of SnI 4 were sealed in an evacuated Pyrex tube. The tube was heated to 650 °C with a rate of 1.4 °C min −1 and kept at 650 °C for 5 h, followed by cooling down to 500 °C with a rate of 0.3 °C min −1 . After the sample, was naturally cooled down to room temperature, the product was washed with hot toluene and acetone for three times to remove the residual mineralizer. Finally, the product was dried under vacuum for further analysis. BP nanosheets were prepared by liquid exfoliation of bulk BP. In detail, 200 mg of bulk BP was dispersed in 500 mL of NMP. The mixture solution was then sonicated in ice water for 8 h. Ice water was used to keep the system at relatively low temperature. Afterwards, the resultant brown suspension was centrifuged at 150 × g for 10 min to remove the residual unexfoliated particles. The supernatant was collected by centrifugation at 11,242 × g for 10 min and washed by a mixture of hexane, chloroform, and ethanol. After been washed for three times, BP nanosheets were dried under vacuum for further use. In a typical synthesis of Au 1 /BP nanosheets, 400 mg of BP nanosheets was finely dispersed in 500 mL of ethanol under N 2 protection. Then, 20 mL of HAuCl 4 aqueous solution (0.203 mM) was injected into the solution containing BP nanosheets through a two-channel syringe pump at room temperature for 4 h under N 2 protection. The product was collected by centrifugation, washed three times with ethanol, and then dried under vacuum. Further ICP-AES result determined that the mass loading of Au was 0.2 wt%. The syntheses of Pt 1 /BP, Rh 1 /BP, and Pd 1 /BP nanosheets with metal loading of 0.2 wt% followed the same method as that of Au 1 /BP nanosheets, despite that H 2 PtCl 4 , RhCl 3 , and Na 2 PdCl 4 were used as precursors, respectively. The syntheses of Au NPs/BP, Pt NPs/BP, Rh NPs/BP, and Pd NPs/BP nanosheets with metal loading of 1.0 wt% followed the method of NaBH 4 reduction. In all, 400 mg of BP nanosheets were finely dispersed in 500 mL of ethanol under N 2 protection. Then, 20 mL of HAuCl 4 (1.02 mM), H 2 PtCl 4 (1.03 mM), RhCl 3 (1.94 mM), or Na 2 PdCl 4 (1.88 mM) aqueous solution was added into BP nanosheets suspension and stirred for 20 min under N 2 protection. In all, 8 mL of NaBH 4 aqueous solution (20 mg/mL) was added into the mixture. After further stirring for 40 min, the samples were collected by centrifugation, washed with ethanol for three times, and then dried under vacuum. Catalytic tests The partial oxidation of methane into methanol was carried out in a 180-mL stainless-steel slurry reactor (Shanghai Yanzheng Experiment Instrument Co., LTD, China). The sapphire window with an irradiation area of 3.14 cm −2 at the top of slurry reactor allows the incidence of light from Xe lamp (PLS-SXE300, PerfectLight, China) into the reactor to participate in the photocatalysis. Full-spectrum light was adopted for catalytic tests. The intensity of irradiation light was determined by a spectroradiometer (PL-MW2000, PerfectLight, China). After the addition of 20 mL of H 2 O and 200 mg of catalysts into a Teflon inlet, the slurry reactor was pressurized with CH 4 (30 bar) and O 2 (3 bar) at room temperature. Then, the slurry reactor was heated to 90 °C and kept for 2 h with stirring at 500 rpm. After completion of the reaction, the slurry reactor was quickly cooled by ice water. The gas-phase was determined by gas chromatographs (Shimadzu GC-2014) equipped with a thermal conductivity detector (TCD) and a flame ionization detector (FID). The liquid phase of the reaction mixture was collected by centrifugation at 14,962 × g for 5 min. 20 μL of DMF was introduced into 0.4 mL of the reaction mixture as an internal standard. In all, 100 μL of the mixture was dissolved in 0.4 mL of DMSO-d 6 to determine the product yields by 1 H NHR spectroscopy. In situ cycles For each cycle, the catalytic reaction was operated under CH 4 (30 bar) and O 2 (3 bar) at 90 °C for 2 h. After cooling down, the product in gas phase was detected by both GC-TCD and GC-FID. 0.4 mL of liquid products were taken for further analysis without open the reactor. Afterwards, the reactor was re-pressured with CH 4 (30 bar) and O 2 (3 bar), followed by being reheated to 90 °C and kept at this temperature for another 2 h. The whole durability test continued for 10 in situ cycles. XAFS measurements XAFS spectra at Au L 3 -edge ( E 0 = 11,919 eV) were performed at BL14W1 beamline of Shanghai synchrotron radiation facility operated at 3.5 GeV under “top-up” mode with a constant current of 220 mA. The XAFS data were recorded under fluorescence mode with a 3 2 − element Ge solid state detector. The energy was calibrated according to the absorption edge of pure Au foil. Athena and Artemis codes were used to extract the data and fit the profiles. For the XANES part, the experimental absorption coefficients as a function of energies μ ( E ) were processed by background subtraction and normalization procedures. This process was reported as “normalized absorption”. For the EXAFS part, the Fourier transformed (FT) data in R space were analyzed by applying the first shell approximation or metallic Au model for the Au–P or Au–Au shell, respectively. The passive electron factors, S 0 [2] , were determined by fitting the experimental Au foil data and fixing the Au–Au CN to be 12, and then fixed for further analysis of the measured samples. The parameters describing the local structure environment including CN , bond distance ( R ) and Debye Waller ( D.W .) factor around the absorbed atoms were allowed to vary during the fit process. In situ DRIFTS measurements In situ DRIFTS experiments were conducted in a cell with a Fourier transform infrared spectrometer and a liquid nitrogen cooled detector. In all, 1 mg of Au 1 /BP was diluted in 200 mg of KBr. As for treatments without CH 4 in the dark (Fig. 3a ), the background spectrum of the sample was acquired after flowing under 1 bar of N 2 with the rate of 20 sccm at 150 °C for 0.5 h, followed by cooling to 90 °C. For the treatment with O 2 , the sample was purged by 1 bar of O 2 with the rate of 10 sccm at 90 °C for 0.5 h, followed by 1 bar of N 2 with the rate of 20 sccm at 90 °C for 0.5 h. The procedure for the treatment with N 2 was similar to that for the O 2 treatment, except for the use of 1 bar of N 2 to replace O 2 . For the treatment with O 2 /H 2 O, 1 bar of O 2 was allowed to bubble in deionized water, followed by flowing into the cell, in order to bring the saturated water vapor into the cell. The sample was purged by the mixed gas containing O 2 and H 2 O with the rate of 10 sccm at 90 °C for 0.5 h, followed by 1 bar of N 2 with the rate of 20 sccm at 90 °C for 0.5 h. The procedure for the treatment with N 2 /H 2 O was similar to that for the treatment with O 2 /H 2 O, except for the use of 1 bar of N 2 to replace O 2 . The procedures for treatments without CH 4 under light irradiation (Fig. 3 b) were similar to those in the dark, except for using Xe lamp (1.2 W) to illuminate the cell. As for treatments with CH 4 in the dark (Fig. 3e ), the sample was pre-treated under 1 bar of O 2 /H 2 O with the rate of 10 sccm at 90 °C for 0.5 h to generate P=O and P–O–P ensembles. Afterwards, the sample was purged by 1 bar of CH 4 with the rate of 10 sccm at 25 °C for 0.5 h to obtain background spectra. In situ DRIFTS spectrum was recorded under 1 bar of CH 4 with the rate of 10 sccm at 90 °C in the dark. The procedure for the treatment with CH 4 under light irradiation (Fig. 3f ) was similar to that in the dark, except for using Xe lamp (1.2 W) to illuminate the cell. Notably, the pre-treatment with O 2 /H 2 O under light irradiation aimed at yielding P=O, P–O–P, and P–OH ensembles. DRIFTS measurements using CO as a probe molecule The background spectrum of the sample was acquired after flowing under 1 bar of N 2 with the rate of 20 sccm at 150 °C for 0.5 h, followed by cooling to 25 °C. Then, 1 bar of 10%CO/Ar with the rate of 10 sccm was allowed to flow into the cell for 20 min. 1 bar of N 2 with the rate of 20 sccm was used to purge out the gaseous CO from the sample cell so that the chemically adsorbed CO species on the samples could be detected. In situ ESR measurements Au 1 /BP nanosheets were dispersed in water pre-saturated with CH 4 and O 2 to detect possible radicals (4 g L −1 ). As for the 1 O 2 trapping-ESR tests, 50 μL of aqueous suspension of samples was mixed with 500 μL of 2,2,6,6-tetramethylpiperidine (50 mM) solution. After being illuminated for 1 min, the mixture was characterized using an ESR spectrometer (JEOL JES-FA200) at room temperature. As for the O 2 − and •OH trapping-ESR tests, similar procedures were adopted except the use of 5,5-dimethyl-1-pyrroline-N-oxide (DMPO) as the spin-trapping agent. TOF calculation The TOF numbers were calculated based following equation (equation 10): 
    [                                             TOF;           = ( n_CH3OH + n_CO2)/( t × n_surface);           = ( n_CH3OH + n_CO2)/( t ×δ× n_metal); = ( n_CH3OH + n_CO2)/( t ×δ× m_cat× w/μ _metal) ]
 (10) In these equations, n CH3OH represents the mole of produced CH 3 OH molecules. t is the reaction time. n surface is the mole of surface metal atoms. δ is the molar ratio of surface atom. n metal is the mole of total metal atoms. m cat is the mass of the catalysts. w is the mass loading of the catalysts. μ metal is the atomic mass. For single atoms, δ = 100%. For NPs, δ was calculated using the following equations (equations 11–13) given by Vannice [29] : 
    [ δ = 6 × 10^7 ×( V_metal/A_metal) ×( 1/d_metal) × 100%;                                                       ]
 (11) 
    V_metal = μ _metal/( ρ _metal× N_A)
 (12) 
    A_metal = 1/n_s
 (13) where V metal is the bulk atomic volume of the metals (cm [3] ), A metal is the area of an atom (cm 2 ), and d is the metal particle size in nm. μ metal is the atomic mass, ρ is the bulk density, and N A is Avogadro’s number. n s is the average site density. The n s of Au, Pt, Rh, Pd were 1.2 × 10 15 , 1.3 × 10 15 , 1.3 × 10 15 , and 1.3 × 10 15 cm −2 , respectively [30] . Thus A metal were calculated as 8.7 × 10 −16 , 8.0 × 10 −16 , 7.5 × 10 −16 , 7.9 × 10 −16 cm 2 . The values of V metal were calculated as 1.7 × 10 −23 , 1.5 × 10 −23 , 1.4 × 10 −23 , 1.5 × 10 −23 cm 3 for Au, Pt, Rh, and Pd, respectively. The average sizes ( d metal ) of NPs were measured to be 6 nm, 5 nm, 4 nm, and 6 nm for Au, Pt, Rh, and Pd, respectively, based on TEM images. Therefore, the values of δ were calculated to be 19.5%, 22.6%, 27.5%, and 18.6% for Au, Pt, Rh, and Pd, respectively. The TOF numbers of Au 1 /BP, Pt 1 /BP, Rh 1 /BP, Pd 1 /BP, Au NPs/BP, Pt NPs/BP, Rh NPs/BP, and Pd NPs/BP nanosheets were calculated as 5.6, 4.5, 1.1, 3.2, 3.3, 0.8, 0.2, and 2.1 h −1 , respectively. Conversion calculation The conversion was calculated based following equation (equation 14): 
    Conversion = ( n_CH3OH + n_CO2)/n_CH4× 100%
 (14) The amount of CH 4 charged into the reactor is calculated from 30 bar of CH 4 at room temperature. The volume of gas is 160 mL, which corresponds to 193.6 mmol CH 4 . The conversion after 2 h was calculated as 0.01%. We chose a low conversion in order to measure the kinetic parameters such as the reaction rate, TOF, and E a , because the temperature, pressure, and concentrations can be regarded as constant throughout the reactor [31] . AQY measurements The apparent quantum yields (AQY) were measured under the irradiation of monochromatic lights at 350, 380, 450, 500, 550, 600, 650, and 765 nm using band-pass filters. The irradiation area was 3.14 cm 2 . The intensities of irradiation light was determined to be 2.1, 4.2, 21.9, 15.6, 19.3, 23.9, 26.0, and 23.9 mW·cm −2 for 350, 380, 450, 500, 550, 600, 650, and 765 nm, respectively. The formation of one methanol molecule only consumes one photo-generated electron during the generation of reactive hydroxyl groups and •OH radicals. The AQY was calculated according to the following equation (equation 15): 
    AQY =	  1 × N_CH3OH/N_photons× 100%
     =	  1 × N_CH3OH× N_A/[W × A × t/(h ×υ )] × 100%
 (15) N CH3OH and N photons represent the number of formed CH 3 OH and the number of incident photons. υ , W , A , and t are the incident light frequency, intensity, irradiation area and time, respectively. N A and h are the Avogadro’s constant and Planck constant, respectively. The AQYs were calculated to be 17.4%, 8.7%, 1.3%, 0.9%, 1.0%, 0.6%, 0.4%, and 0.4% for 350, 380, 450, 500, 550, 600, 650, and 765 nm, respectively. TPSR-MS measurements In all, 100 mg of Au 1 /BP nanosheets were pre-treated by being immersed in 5 mL 18 O-labeled water (H 2 18 O) under O 2 ( 32 O 2 ) flow in the dark or under light irradiation (1.2 W) at 90 °C for 0.5 h. The treated samples were dried under vacuum, followed by being loaded into the quartz tube for further measurement. For TPSR-MS measurements, the pre-treated samples were heated in helium with a gas-flow rate of 20 mL min −1 at 200 °C for 1 h. After cooling down to 50 °C, the gas was switched to 10% CH 4 /Ar (v/v) with a gas-flow rate of 20 mL min −1 . Mass spectral responses were collected from 50 to 300 °C at 5 °C min −1 . We detected the mass numbers (m/z) of 33 for CH 3 18 OH, 31 for CH 3 16 OH, 19 for H 2 18 O, 17 for H 2 16 O, 48 for C 18 O 2 , 46 for C 18 O 16 O, and 44 for C 16 O 2 . DFT calculations Spin-polarized DFT calculations were performed through Vienna ab initio simulation package [32] , [33] . The electron-ion interaction was described via the projector augmented wave method [34] . The exchange-correlation interaction was described via the optB86b-vdW functional [35] . The plane-wave basis set was used to solve the Kohn–Sham equations, whereas the kinetic energy cutoff was 400 eV. In our calculations, a 12-Å vacuum layer and a single layer of BP with (3 × 3) supercells were constructed to simulate Au 1 /BP nanosheets. All the atoms were relaxed during the structure optimization until the maximum force on any ion was less than 0.02 eV Å −1 . The (4 × 3 × 1) k -point mesh was used to sample the Brillouin zone. The climbing-image nudged elastic band method was used to identify the transition states until the maximum force on any ion was less than 0.05 eV Å −1 [36] .